Origin of pressure-induced crystallization of Ce75Al25metallic glass Phase transitions in amorphous alloys under pressure are an important fundamental problem. Here we report on a first-principles study that reproduces the recently discovered pressure-induced crystallization of amorphous Ce 100− x Al x ( x <25) alloys and reveals an atomistic transformation mechanism. Contrary to common belief, pressure-induced devitrification of an amorphous Ce–Al alloy is not due to the Ce 4 f delocalization that is expected to bring the size of Ce atoms closer to that of Al atoms. Our theoretical results show that the Bader volume of Ce is always larger than that of Al. A continuous increase in the relative Ce/Al Bader volume leads to favourable conditions for forming a close-packed structure at high pressure. The results also show that the Hume–Rothery rules are not applicable to describe the structures of substitutional alloys at high pressure. This study provides a new perspective on the electron distribution in lanthanide alloys under the application of pressure. Understanding the microscale structural evolution that takes place as a disordered liquid transitions into to an intermediate-range-ordered glass and eventually a long-range-ordered crystal is of fundamental importance [1] , [2] . Pressure is a versatile and controllable thermodynamic variable that can be used to alter the electronic structure and properties of materials. Compression provides a means to study continuous changes in short-, intermediate- and long-range structural ordering. Recently, neutron and X-ray inelastic scattering experiments have shown that, under pressure, the atomic dynamics of a liquid share many similarities with that of its glass and solid phases [3] , suggesting a possible connection in their structural ordering. This study is motivated by the phenomenon that disordered Ce 100− x Al x metallic glasses with a stoichiometry corresponding to x <25 can be ordered by compression [4] , [5] , [6] . Although glasses are common materials and have been well studied, their structures are not fully understood. The observation described in this work opens a new dimension in the field of glass science. In particular, we aim to answer the question of whether ordering by compression indicates an inherent ‘hidden’ order in amorphous solids, or is simply a manifestation of a change in the electronic structure. A fundamental understanding of the underlying mechanism will help to clarify the progressive development of these systems from short- to long-range order. It is also surprising that these phase transitions were observed in Ce-based amorphous alloys, which were believed to have already attained the maximum coordination number [4] , [5] , [6] , [7] , [8] , [9] , [10] , [11] , [12] , [13] , [14] , [15] , [16] , [17] , [18] , [19] . The most thoroughly exprimentally studied system is amorphous ( a -) Ce 75 Al 25 metallic glass, which transforms into a crystalline substitution solid solution with a face-centred cubic (FCC) structure under quasi-hydrostatic conditions, 25 GPa and ambient temperature [4] , [5] , [6] . It is generally accepted, albeit without sound theoretical justification, that this structural transformation is the consequence of pressure-induced Ce 4 f to 5 d hybridization that results in a smaller size difference between Ce and Al, thus favouring a close-packed structure. However, this conjecture has never been quantitatively scrutinized. By contrast, it is already well known that for main group metals and metal alloys under pressure, the transfer of valence electrons into interstitial sites in the condensed phases (liquid and crystalline) is a common phenomenon. There is therefore no guarantee that the size of the Al atom will be modified concomitantly following a similar trend. Thus, it is imperative to understand whether the structural phase transition is simply driven by a geometric effect. If not, the roles that the electronic structure, Ce and Al atomic volume and electronegativity play in the Ce 75 Al 25 amorphous alloy under pressure should be understood. To answer these questions, we have performed a detailed theoretical investigation of this interesting process. Static electronic structure calculations and ab initio molecular dynamics (MD) simulations have been performed to study the unusual pressure-induced amorphous–crystalline transformation in Ce 75 Al 25 metallic glass. It was found that, contrary to the prevailing belief, the phase transition is not caused by Ce 4 f –5 d hybridization [4] , [5] . Instead, the crystallization is driven by a steric effect that arises when the atomic size of Ce becomes dominant in the Ce-rich glasses, which leads to the formation of a cubic close-packed structure at high pressure. This is the consequence of the change in local structure and arrangement of randomly distributed small Al aggregates that are modified by continuous back charge transfer from Al to Ce. The theoretical results presented in this work provide an atomistic explanation of the amorphous–crystalline transition in a -Ce 75 Al 25 . The novel charge transfer process discovered in this study also provides new insight into the charge delocalization and volume reduction that should be common to all lanthanide alloys at high pressures. Bader atomic volume of ordered crystalline Ce 3 Al It is generally assumed that the atomic size of a Ce atom is much larger than that of an Al atom under ambient conditions. Under compression, as Ce is expected to undergo a 4 f –5 d transition in which a localized 4 f electron is ‘promoted’ to the itinerant 5 d orbital, the atomic size is greatly reduced, making it more comparable to Al. If the alloying atoms have similar size, close-packed structures (that is, FCC or hexagonal close packing (HCP)) are preferred. Therefore, how the concept of atomic size can be uniquely defined in a disordered system and the way it evolves with the application of external pressure is central to the understanding of the amorphous-crystal transformations in Ce–Al alloys. Unfortunately, the choice of atomic sizes in the condensed phase is subject to ambiguity. The general approach of partitioning the charge inside the Wigner–Seitz (WS) cell is often not appropriate for high-pressure structures because a fixed-radius WS cell for each atom is used, making comparisons at different pressures ambiguous. An unbiased approach is to employ the Bader atom-in-molecule method [20] , in which atomic volume is uniquely defined by the charge-density topology as the region bound by zero-flux surfaces. It is well known that the traditional functionals used in density functional theory calculations are inadequate to describe localized d and f valence orbitals in transition or rare-earth atoms [21] , [22] . The first task is therefore to devise a computational scheme that ensures that the theoretical results are reliable over a broad pressure range, after exploring several approaches. As will be shown and validated in the Methods section, calculations that use potentials with localized and delocalized 4 f orbitals agree well with experimental results at low and high pressure, respectively. We circumvented this problem by adopting an ad hoc approach that treats the environmental dependence of the Ce 4 f orbitals with different projected augmented potentials (PAWs). The starting point of the discussion is to characterize the crystal and electronic structure of a known crystalline alloy, Ce 3 Al. This ordered alloy has a cubic structure and is stable under ambient conditions. Employing Bader volumes to define atomic size, Al atoms were calculated to be larger than Ce atoms in crystalline Ce 3 Al at low pressure, regardless of the PAW potentials and density functional used in the calculations ( Supplementary Figs 1 and 2 ). Aluminium has a larger Bader volume at ambient pressure because the alloy formation is driven by charge donation from the more electropositive Ce (electronegativity χ of 1.12 on the Pauling scale) to the more electronegative Al ( χ =1.61). This observation contradicts the perception that Ce is larger than Al. More surprisingly, the Bader volume of Al decreases more rapidly than that of Ce with increasing pressure and eventually becomes the smaller of the two ( Supplementary Fig. 1 ). Crystallization of a -Ce 75 Al 25 structures under pressure Having demonstrated the potential shortcomings of the assignment of atomic sizes, we will now analyse the a -Ce 75 Al 25 structures obtained from ab initio MD calculations. The calculated structural factor at ambient pressure shown in Fig. 1a is in good agreement with the experimental value, indicating that a reasonable amorphous structure has been generated. The Atomic Cluster Alignment method [23] was used to determine the degree of topological ordering. In this method, cluster regions extracted from the simulated structure are aligned so that local structure information is preserved and the resulting dominant cluster feature can be examined visually. Visual identification has the advantage of being direct, and it is intuitively more appealing compared with the conventional structure characterization methods that rely on the calculations of specific order parameters. The local structures obtained from the Atomic Cluster Alignment analysis of a -Ce 75 Al 25 at selected pressures are depicted in Fig. 2 . The local structural order is clearly very different between 0 GPa and 25 or 38 GPa ( vide infra ). At 0 GPa, the aligned clusters exhibit weak short-range order, indicating a highly disordered structure. Although a much clearer short-range order is observed at 25 GPa, the aligned cluster shows no translational periodicity. Thermal annealing at 800 K for 30 ps did not result in a crystalline solid. In comparison, the aligned clusters evaluated at 38 GPa show a highly symmetric feature, indicating that a long-range topological order has been established. The resulting structure after short annealing shows an unambiguously ordered Ce arrangement interspersed with the Al neighbours ( Fig. 3 ). A comparison of the energies of the alignment templates ( Fig. 2d–f ) unequivocally shows FCC packing of the atomic structure. The appearance of the FCC ordering is also reflected in the evolution of the bond-angle distribution as a function of pressure ( Supplementary Fig. 3 ). It is clear that the two major distributions shift to 60 and 120 degrees with increasing pressure, which is characteristic of FCC packing. In agreement with experimental results [4] , the ordered structure is a substitutional alloy (that is, the Al atoms occupy the lattice sites, rather than the interstitial sites, see Fig. 3b and Supplementary Fig. 4 ). Therefore, an amorphous-to-crystalline phase transition has been successfully reproduced by our theoretical calculations. 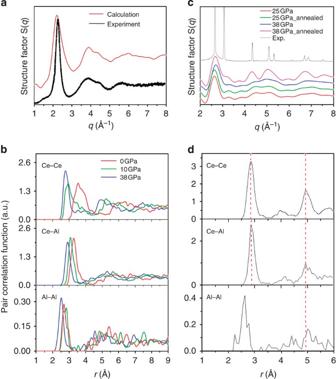Figure 1: Structural analysis of Ce75Al25metallic glass. (a) Comparison of the calculated and experimental structure factorS(q) at 0 GPa. (b) PCF at selected pressures. (c) Comparison of the calculatedS(q) at different pressures together with the experimental crystalline phase. (d) PCF annealed at 38 GPa. The dashed lines are provided to guide the eye. Figure 1: Structural analysis of Ce 75 Al 25 metallic glass. ( a ) Comparison of the calculated and experimental structure factor S ( q ) at 0 GPa. ( b ) PCF at selected pressures. ( c ) Comparison of the calculated S ( q ) at different pressures together with the experimental crystalline phase. ( d ) PCF annealed at 38 GPa. The dashed lines are provided to guide the eye. 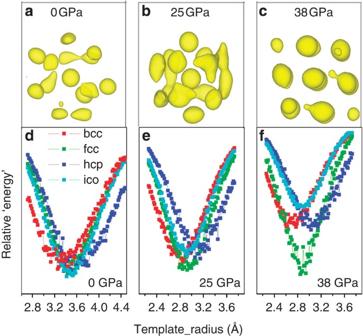Figure 2: Cluster alignment results ofa-Ce75Al25structure at selected pressures. (a–c) Aligned clusters from structures at 0, 25 and 38 GPa, respectively. (d–f) Energies of alignment templates at 0, 25 and 38 GPa, respectively. Full size image Figure 2: Cluster alignment results of a -Ce 75 Al 25 structure at selected pressures. ( a – c ) Aligned clusters from structures at 0, 25 and 38 GPa, respectively. ( d – f ) Energies of alignment templates at 0, 25 and 38 GPa, respectively. 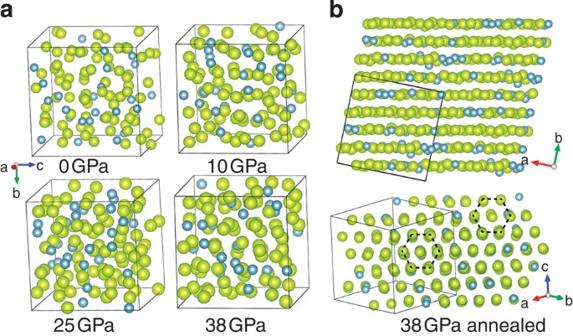Figure 3: Snapshots ofa-Ce75Al25structures. (a, left panel) Structures at selected pressures. (b, right panel) The annealed structure at 38 GPa. Note that the honeycomb packing of the FCC lattice is clearly visible down the [111] direction. Full size image Figure 3: Snapshots of a -Ce 75 Al 25 structures. ( a , left panel) Structures at selected pressures. ( b , right panel) The annealed structure at 38 GPa. Note that the honeycomb packing of the FCC lattice is clearly visible down the [111] direction. Full size image To gain insight into the crystallization process, atomic pair-correlation functions (PCFs; Fig. 1b,d ) were analysed. We found that the Al atoms are not evenly distributed in the structure but instead tend to aggregate, forming small clusters. The calculated average nearest Al–Al neighbour distance of 2.7 Å in the theoretical glass structure confirms the suggestion made from previous experimental studies [5] , [12] . A Bader charge analysis shows that at 0 GPa each Al atom in the glass structure gains an average of 1.05 e from the Ce atoms. This is 0.30 e less than in the case of crystalline Ce 3 Al, for which each Al atom gains 1.35 e from the Ce atoms as the Bader volume of Al becomes closer to that of Ce. At pressures of over 10 GPa, the trend in the change of the atomic volume with pressure in a -Ce 75 Al 25 is similar to that of crystalline Ce 3 Al, for which the Bader volume of Al atoms decreases faster than that of Ce because of electron back donation from Al to Ce ( Fig. 4a,b ). Qualitatively, the predicted electron back donation is also reflected in the atomic charge differences calculated in the WS atomic cells ( Supplementary Fig. 5 ). Consequently, the Bader atomic volume ratio V Ce / V Al becomes larger at high pressure. The theoretical evidence contradicts the hypothesis [4] , [5] , [6] that a favourable condition for the formation of a substitution alloys is the reduction in the Ce atomic volume to bring it closer to that of Al. The projected density of states ( p -DOS) shown in Supplementary Fig. 6 reveals that there is no significant hybridization of the Ce 4 f and Al 2 p orbitals. This also indicates that the delocalized 4 f electrons do not contribute directly to the structural stability of the glass. The PCF calculated at different pressures ( Fig. 1c ) shows that the first Ce–Ce nearest neighbour peaks at 0 and 10 GPa are very broad, indicating a structurally diverse local environment. By contrast, at 38 GPa the first Ce–Ce peak in the PCF becomes narrower, suggesting that the average local structures are now much more similar. In addition, the closest Ce–Ce distance has been shortened and is closer to the first peak of the Ce–Al pair. Changes in the local environment at high pressure are obvious from the observed change in the Bader volumes ( Fig. 4 ). At 0 GPa, the mean Bader volume difference ( V Ce −V Al ) /V Al is 13%, and the spread (deviation from the mean) spans a fairly large range of 23–39 Å 3 . At 38 GPa, the crystalline phase transition emerges and the spreads in the Ce and Al Bader volumes are now much smaller, even though the difference has increased to 40%. The establishment of long-range order is evident from the nearly identical peak positions corresponding to Ce–Ce, Ce–Al and even Al–Al (except the nearest neighbour peak) PCFs. The sample annealed at 800 K shows an even narrower Bader volume fluctuation of ca . 1 Å 3 per atom and exhibits a much higher degree of crystallinity. This fact is reflected in the structure factors and the structures, which are shown in Figs 1c and 3b , respectively. Despite minor defects due to Al aggregates, the calculated structure factor of the annealed structure at 38 GPa exhibits Bragg peaks that match well with the experimentally obtained diffraction pattern. 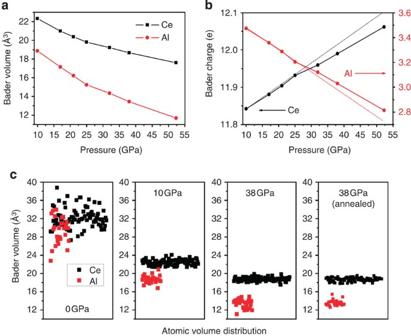Figure 4: Bader topological analysis ofa-Ce75Al25at different pressures. (a,b) The Bader volume and charge, respectively. (c) Bader atomic volume distribution for all of the atoms ina-Ce75Al25at selected pressures. It should be noted that the structure at 0 GPa was generated using the Ce_11 potential, whereas all of the compressed structures were generated using the Ce_12 potential. Figure 4: Bader topological analysis of a -Ce 75 Al 25 at different pressures. ( a , b ) The Bader volume and charge, respectively. ( c ) Bader atomic volume distribution for all of the atoms in a -Ce 75 Al 25 at selected pressures. It should be noted that the structure at 0 GPa was generated using the Ce_11 potential, whereas all of the compressed structures were generated using the Ce_12 potential. Full size image A closer examination of the Bader charge and volume of an individual Al atom in a -Ce 75 Al 25 reveals that the Al aggregates play a vital role in the devitrification process. 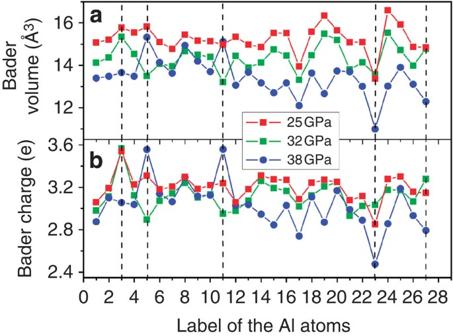Figure 5: Bader analysis of individual Al atoms in a-Ce75Al25. (a) Bader volume analysis. (b) Bader charge analysis. Several anomalies are marked with dashed lines. The coloured solid lines are provided to guide the eye. Figure 5 compares the volume and charge distribution of an individual Al atom at 25, 32 and 38 GPa. Several anomalies were observed after the transition at 38 GPa. For example, there are noticeable differences in the behaviour of Al atom number 3, 5, 11, 23 and 27 compared with the rest. The charges on Al number 5 and 11 were increased by ca . 0.5 e compared with those at 32 GPa, and Al number 3, 23 and 27 concomitantly decreased by 0.4 e . Inspection of the structure shows that these ‘anomalous’ Al atoms are clustered to each other, forming small aggregates ( Fig. 6 ). Before crystallization, the size of the cluster is comparatively large and prohibits the surrounding Ce atoms from adopting a more regular closed packing configuration. At 38 GPa, one of the Al atoms in this cluster has migrated into another layer of Ce atoms, with the result that the ‘volume’ occupied by the aggregate is reduced, facilitating the packing into an FCC-like structure ( Fig. 6c ). Figure 5: Bader analysis of individual Al atoms in a-Ce 75 Al 25 . ( a ) Bader volume analysis. ( b ) Bader charge analysis. Several anomalies are marked with dashed lines. The coloured solid lines are provided to guide the eye. 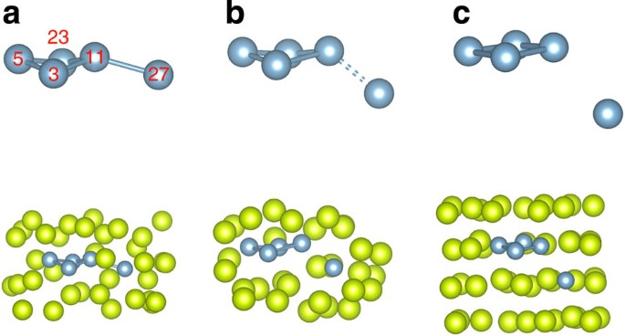Figure 6: Al clusters and their local structure at selected conditions. (a) After annealing at 800 K, 32 GPa, (b) 38 GPa and (c) 38 GPa. The grey and yellow balls are Al and Ce atoms, respectively. Full size image Figure 6: Al clusters and their local structure at selected conditions. ( a ) After annealing at 800 K, 32 GPa, ( b ) 38 GPa and ( c ) 38 GPa. The grey and yellow balls are Al and Ce atoms, respectively. Full size image Because no amorphous-to-crystalline transition was observed in an a -La 75 Al 25 alloy up to ~40 GPa(ref. 24 ), to validate the computational results and the discussions presented above, we have performed similar MD calculations on an a -La 75 Al 25 alloy. In agreement with the experimental results, no crystallization was found at least up to 52 GPa. The calculations showed that on average each Al atom in the a -La 75 Al 25 alloy accepted ~0.2 e more than in the a -Ce 75 Al 25 alloy. Thus, the larger sizes of the Al aggregates are not comparable to the vacant sites of the La atoms, preventing a close-packed structure. In conclusion, ab initio MD calculations have been performed to characterize the pressure-induced amorphous-to-crystalline phase transition in a -Ce 75 Al 25 . The experimental amorphous-to-crystalline phase transition was correctly reproduced. The transfer of Ce 4 f electrons to the more delocalized 5 d orbital only contributes to the volume collapse that takes place at very low pressures, that is, between 1.5 and 5.0 GPa (ref. 14 ). Therefore, it is not responsible for the transformation to the crystalline phase occurring at 25 GPa. It is shown that the general concept of the relative size of atoms under ambient conditions is not applicable to describe the structure at high pressure. By contrast, the Bader atomic volumes of Ce and Al atoms were found to be similar in the amorphous phase under ambient pressure. Compression does not decrease the Bader volume difference between Ce and Al. Conversely, the V ce / V Al Bader volume ratio actually increases with pressure, and at 38 GPa the Ce Bader volume is 40% larger than that of Al. As a result, the amorphous–crystalline transformation is driven by the packing of the dominant Ce into an FCC structure, which is the result of a sudden change of the charge transfer from Al to Ce atoms. The present theoretical investigation suggests the following mechanism. Under ambient conditions, the broad Bader atomic volume distributions of Ce and Al atoms indicate that the alloy is a random glass. As the pressure is increased to 5 GPa, the anticipated Ce 4 f –5 d transition takes place. Unlike crystalline Ce 3 Al, in which the Al atoms are separated far from each other in the crystal structure, the presence of Al aggregates in the glass structure reduces electron transfer from Ce to Al. It is important to note that at 38 GPa, the Bader charges are almost the same in the respective atoms, indicating that there is very little charge transfer occurring. However, the Bader atomic radius of Ce at this pressure is 11% larger than that of Al, and the structure is crystalline. These observations bring up the possibility that pressure-induced amorphous–crystalline transformations may obey the traditional Hume–Rothery rules, which state that (a) the difference in the atomic radii of the two species is less than 15% and (b) their electronegativity should be similar. However, this possibility can be shown to be incorrect because the Ce/Al Bader volume ratio and charge difference between Ce and Al continue to increase beyond the transition pressure, whereas the structure remains as a substitutional alloy without transforming into another structure. In retrospect, it is not surprising that the Hume–Rothery rules are inapplicable at high pressure. These empirical rules use the atomic volumes of elemental solids under ambient conditions and do not account for changes in chemical bonding when the system is compressed. By contrast, as the Bader atomic volumes are determined by the electron-density topology, such changes are considered explicitly for alloys at high pressures. It has been shown in this study that the Al atoms are not randomly distributed in the alloy glass structure. The formation of Al aggregates prevents a close-packed structure from forming at low pressure. At sufficiently high pressure, the Al aggregates deform, and some of the Al atoms migrate into neighbouring Ce planes. This helps to reduce the physical size of the aggregates and to allow more efficient close packing of the majority of the Ce atoms. The mechanism revealed here also explains the experimental observation that amorphous–crystalline transformations occur only in Ce–Al metallic glasses with low Al concentrations (<25 at. %) [6] . Upon increasing the Al concentration, although the size of Ce remains larger than that of Al at high pressure, the formation of many Al aggregate defects prevents close packing. It is likely that an Al concentration of <25 at. % may be the threshold for the pressure-induced crystallization to occur in the studied pressure range. This study gives a new perspective on how valence electrons are distributed under extreme pressure conditions in a metallic glass and provides an atomistic mechanism of the pressure-induced devitrification of amorphous alloys. Validation of the Ce potentials on crystalline Ce 3 Al structures Many studies have shown that it is challenging to correctly reproduce the equations of state (EOS) for crystalline rare-earth elements and compounds over a broad pressure range. To circumvent this problem, the GGA+ U method, which includes an on-site Coulomb repulsion interaction ( U ), has been used to describe the electronic structure of Ce–Al alloys near ambient pressure. In such structures, the Ce 4 f electrons are localized. However, the assumption of a constant U may not be valid over a broad pressure range as the value may change with the nature of the 4 f orbitals [22] . Another strategy is to employ a hybrid functional by adding a portion of exact exchange into the exchange-correlation energy functional. The Heyd–Scuseria–Ernzerhof (HSE) [25] exchange-correlation functional has been demonstrated to yield comparable results with the more rigorous correlated methods and may be used as a benchmark. This functional is computationally too demanding for amorphous structures with a large number of atoms. An ad hoc approach is to treat the Ce 4 f orbitals differently depending on their chemical environment by using different pseudopotentials. Under ambient conditions, when the Ce 4 f electron is localized, an 11-electron (Ce_11)-PAW [26] explicitly excluding the 4 f orbital in the valence with configuration 5 s 2 5 p 6 5 d 1 6 s 2 can be used. At high pressure, the Ce 4 f electron is transferred to the 5 d orbital and the system is metallic. Therefore, a 12-electron (Ce_12) PAW with an electronic configuration of 5 s 2 5 p 6 4 f 1 5 d 1 6 s 2 can be used [4] . The arbitrary division into two different regimes, that is, low and high pressure, that are treated with different PAW potentials is not ideal; however, this procedure was employed previously for the amorphous-to-crystalline phase transition in a -Ce 75 Al 25 at 25 GPa and seems to provide reasonable agreement with experiments [5] . The concern in this case is to validate this procedure for crystalline Ce–Al alloys, particularly at low pressures, to determine whether it could be applied to generate low-pressure Ce–Al glass structures. For this purpose, the EOS and electronic structure of the known FCC intermetallic Ce 3 Al (Pm-3 m) were calculated with Ce_11, Ce_12 and Ce_12+ U ( U =5.6 eV (ref. 12 )) PAW potentials and the Ce_12+HSE functional including spin-polarized calculations. The PAW formalism of density functional theory, as implemented in the Vienna ab initio simulation package, was used [27] , [28] . The generalized gradient approximation as described in ref. 29 was employed to describe the exchange-correlation density function. Electron orbitals were expanded in a plane wave basis set using an electron-density cutoff of 400 eV. Calculations with the Ce_12+ U and Ce_12+HSE PAW potentials predicted a high spin state and cubic lattice constants of 4.919 and 4.960 Å, respectively. These values are comparable to the experimental value of 5.015 Å (ref. 30 ; Supplementary Fig. 7a ). Unexpectedly, the Ce_11 calculations also yield a reasonable unit cell size of 4.993 Å. The Ce_12+HSE calculations predicted an iso-structural transition to a dense metallic phase with a large volume reduction at 20–25 GPa. As revealed from the atomic occupation analysis ( Supplementary Fig. 7b ), this transition is caused by the transfer of an electron from the Ce 4f to 5d orbital. The EOS from the HSE calculation agrees well with both the Ce_11 and Ce_12+ U PAWs at low pressures (<5 GPa), whereas it agrees much better with the Ce_12 method at high pressures (>25 GPa) because Hartree exchange becomes less important in the metallic structure. The agreement between the HSE, Ce_12+ U and Ce_11 PAW results are also observed in the calculated Bader volumes ( Supplementary Fig. 1 ). To further validate the Ce_11 and Ce_12 potentials, a comparison of the EOS to the experimental work in ref. 4 was also performed ( Supplementary Fig. 7c ). We find that Ce_11 result agrees reasonably well with the experiment results obtained on Ce 3 Al (P6 3 /mmc) at ambient pressure before the 4 f delocalization. However, the Ce_12 result agrees extremely well with experiment results on the FCC alloy measured in the high-pressure region. MD calculations of the a -Ce 75 Al 25 structures Ab initio MD (AIMD) calculations in the canonical ensemble [31] were performed on models containing 108 atoms [32] , [33] . Only the Γ point was used for Brillouin zone sampling. The Nose–Hoover thermostat was used to control the temperature [31] . An ambient a -Ce 75 Al 25 structure model was prepared by melting crystalline Ce 3 Al at 2,000 K (melting point ~900 K) using MD calculations with the Ce_11 PAW potential. The system was then cooled in steps to 300 K and annealed for 18 ps. The calculated and observed structure factors ( S ( q )) for a -Ce 75 Al 25 at ambient pressure are compared in Fig. 1a , which shows that all of the major features are reproduced by the theoretical model. Significantly, Al aggregates consisting of a few Al atoms were found to be distributed evenly over the glass structure. Above 10 GPa, the glass structures were obtained from compressing the low-pressure phase using the Ce_12 PAW potential. At each selected pressure point, the structure was again annealed for at least 18 ps. How to cite this article: Wu, M. et al . Origin of pressure-induced crystallization of Ce 75 Al 25 metallic glass. Nat. Commun . 6:6493 doi: 10.1038/ncomms7493 (2015).